FoxP3+regulatory T cells promote influenza-specific Tfh responses by controlling IL-2 availability Here, we test the role of FoxP3 + regulatory T cells (Tregs) in controlling T follicular helper (Tfh) and germinal centre (GC) B-cell responses to influenza. In contrast to the idea that Tregs suppress T-cell responses, we find that Treg depletion severely reduces the Tfh cell response to influenza virus. Furthermore, Treg depletion prevents the accumulation of influenza-specific GCs. These effects are not due to alterations in TGFβ availability or a precursor–progeny relationship between Tregs and Tfh cells, but are instead mediated by increased availability of IL-2, which suppresses the differentiation of Tfh cells and as a consequence, compromises the GC B response. Thus, Tregs promote influenza-specific GC responses by preventing excessive IL-2 signalling, which suppresses Tfh cell differentiation. T follicular helper cells (Tfh) cells are specialized CD4 + T cells that provide help to B cells via the expression of CD40 ligand and IL-21 (refs 1 , 2 , 3 , 4 ), factors that promote B-cell proliferation, isotype switching, germinal centre (GC) formation and the differentiation of memory B cells and long-lived plasma cells [2] , [3] , [4] , [5] . Tfh cells are distinguished by expression of the chemokine receptor, CXCR5, the inhibitory receptor, PD-1, and the transcription factor, Bcl6, which is the signature transcription factor of the Tfh lineage [4] , [6] , [7] , [8] . Mice in which Bcl6 is eliminated from the T cell lineage fail to develop Tfh cells, do not form GCs and have defects in memory B cells and long-lived plasma cells [6] , [7] , [8] , [9] . The differentiation of Tfh cells is governed by a variety of cellular and molecular interactions that together enforce the expression of Bcl6 and repress the expression of competing transcription factors, particularly BLIMP-1 (refs 3 , 4 , 6 , 10 ). For example, signalling by IL-2 through the IL-2Rα (CD25) on CD4 + T cells inhibits the formation of Tfh by preventing Bcl6 expression via the STAT5 pathway [10] , [11] , [12] , [13] . As a consequence of prolonged IL-2 signalling, Tfh cells do not develop and the development of GCs and long-lived plasma cells is impaired [11] . Thus, the factors that control the physiological availability of IL-2 are likely to regulate Tfh development and the ensuing B-cell response. Whereas IL-2 signalling inhibits the development of Tfh cells, it also promotes the generation, maintenance and function of FoxP3-expressing CD4 + regulatory T cells (Tregs) [14] , [15] , which suppress self-reactive T cells and contribute to the maintenance of peripheral tolerance [15] , [16] , [17] , [18] . Importantly, Tregs constitutively express CD25 and compete with other T cells for available IL-2 (refs 16 , 19 , 20 , 21 , 22 ). Although IL-2 deprivation is proposed to be an important mechanism by which Tregs suppress effector T-cell responses [19] , [20] , [21] , [23] , this same mechanism may paradoxically promote Tfh responses, as IL-2 is a potent negative regulator of Tfh differentiation [10] , [11] , [12] , [13] . However, most studies suggest that Tregs, particularly the CXCR5-expressing T follicular regulatory (TFR) cells [24] , [25] , suppress Tfh and GC B-cell responses [24] , [25] , [26] , [27] , [28] , [29] . In fact, mice with natural or targeted mutations in FoxP3 fail to develop Tregs and spontaneously accumulate autoreactive Tfh and GC cells [25] . Despite their reputation as suppressor cells, Tregs may also promote antigen-specific B-cell responses under some circumstances [24] . In support of this idea, adoptively transferred FoxP3 + Tregs can convert to Tfh in Peyer’s patches and promote B-cell responses to intestinal antigens [30] . Similarly, Tregs promote systemic IgG and mucosal IgA antibody responses following mucosal immunization with protein antigens and cholera toxin [31] . Thus, in addition to suppressing B-cell responses to autoantigens, Tregs may also help B-cell responses to foreign antigens under some circumstances. However, the mechanisms underlying the potential B-cell helper activity of Tregs are incompletely understood. Here, we show that Treg depletion compromises influenza-specific GC responses. Treg depletion also impairs the differentiation of influenza-specific Tfh cells, while increasing the number of IFNg and IL-2-producing effector CD4 + T cells (Teff). Consistent with increased IL-2 production in Treg-depleted animals, CD25 expression is sustained on influenza-specific CD4 + T cells. The loss of Tfh following Treg depletion is not due to a precursor–progeny relationship between FoxP3-expressing cells and Tfh or the lack of TGFβ. Instead, Tregs favour influenza-specific Tfh responses by regulating the availability of IL-2, a potent suppressor of Tfh differentiation. Our findings offer a new perspective for how Tfh and GC responses are controlled and reveal an unexpected, non-suppressive function of Tregs. FoxP3 + cell depletion impairs GC response to influenza To test whether Tregs influenced the GC B-cell response to influenza virus, we intranasally infected C57BL/6 (B6) and FoxP3-DTR [32] mice with influenza A/PR8/34 (PR8), treated them with diptheria toxin (DT) on days 0, 4 and 7 and determined the frequency ( Fig. 1a ) and number ( Fig. 1b ) of FoxP3 + CD4 + Tregs as well as the frequency ( Fig. 1c ) and number ( Fig. 1d ) of CD19 + PNA hi CD38 lo CD138 − GC B cells in the mediastinal lymph nodes (mLNs) on day 10. As expected, Tregs were efficiently depleted in DT-treated FoxP3-DTR mice ( Fig. 1a,b ). Surprisingly, however, both the frequency ( Fig. 1c ) and number ( Fig. 1d ) of total GC B cells were also reduced in Treg-depleted mice. 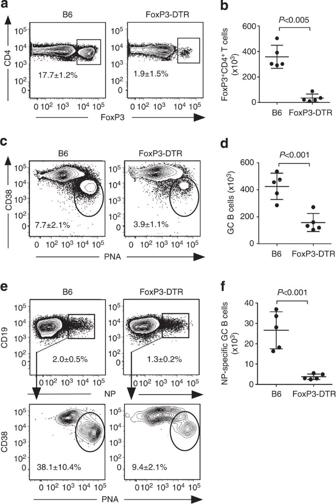Figure 1: Treg depletion compromises GC B-cell responses to influenza. (a–f) B6 and FoxP3-DTR mice were infected with PR8, administered DT on days 0, 4 and 7 after infection and cells from the mLN were analysed on day 10. The frequency (a) and number (b) of CD4+T cells that expressed FoxP3 were determined by flow cytometry. The frequency (c) and number (d) of CD19+CD138−PNA+CD38loGC B cells was determined by flow cytometry. The frequency of NP-specific CD19+B cells (e, top row) and the frequency of NP-specific CD19+PNA+CD38loGC B cells (e, bottom row) were determined by flow cytometry. (f) The number of NP-specific CD19+PNA+CD38loGC B cells was calculated. Data in all panels are representative of five independent experiments (mean±s.d. of five mice).P-values were determined using a two-tailed Student’st-test. Figure 1: Treg depletion compromises GC B-cell responses to influenza. ( a – f ) B6 and FoxP3-DTR mice were infected with PR8, administered DT on days 0, 4 and 7 after infection and cells from the mLN were analysed on day 10. The frequency ( a ) and number ( b ) of CD4 + T cells that expressed FoxP3 were determined by flow cytometry. The frequency ( c ) and number ( d ) of CD19 + CD138 − PNA + CD38 lo GC B cells was determined by flow cytometry. The frequency of NP-specific CD19 + B cells ( e , top row) and the frequency of NP-specific CD19 + PNA + CD38 lo GC B cells ( e , bottom row) were determined by flow cytometry. ( f ) The number of NP-specific CD19 + PNA + CD38 lo GC B cells was calculated. Data in all panels are representative of five independent experiments (mean±s.d. of five mice). P -values were determined using a two-tailed Student’s t -test. Full size image To determine whether Treg depletion prevented the accumulation of influenza-specific GC B cells, we used fluorochrome-labelled recombinant influenza nucleoprotein (NP) tetramers [11] to identify NP-specific GC B cells in Treg-depleted and control mice ( Fig. 1e,f ). We found that both the frequency ( Fig. 1e ) and number ( Fig. 1f ) of NP-specific GC B cells were decreased in Treg-depleted mice. Taken together, these data suggested that FoxP3 + cells promote, rather than inhibit, the generation or maintenance of influenza-specific GC B cells. FoxP3 + cell depletion impairs Tfh cell response to influenza As GC B-cell responses are dependent on help from CD4 + T cells [3] , we next characterized the CD4 + T cells responding to influenza in the mLNs ( Fig. 2a,b ) and lungs ( Fig. 2c,d ) of B6 mice infected 10 days previously. We found that the NP-specific CD4 + T-cell population in the mLN could be separated into two major subsets based on the expression of PD-1 and CXCR5 ( Fig. 2a ). In addition, we found that the NP-specific PD-1 hi CXCR5 hi CD4 + T cells expressed more Bcl6 than the NP-specific PD-1 lo CXCR5 lo CD4 + T cells ( Fig. 2b ). We next characterized the NP-specific CD4 + T-cell response in the lungs and found that the vast majority of NP-specific CD4 + T cells were PD-1 lo CXCR5 lo ( Fig. 2c ) and failed to upregulate Bcl6 ( Fig. 2d ). Thus, we designated the NP-specific Bcl6 hi PD-1 hi CXCR5 hi cells as NP-specific Tfh cells, which were confined to the mLN, whereas we designated the NP-specific Bcl6 lo PD-1 lo CXCR5 lo cells as NP-specific Teff, which we found in both the mLN and lung. As expected, the total number of NP-specific Tfh cells in the mLN increased after influenza infection and peaked around day 7 ( Fig. 2e ). 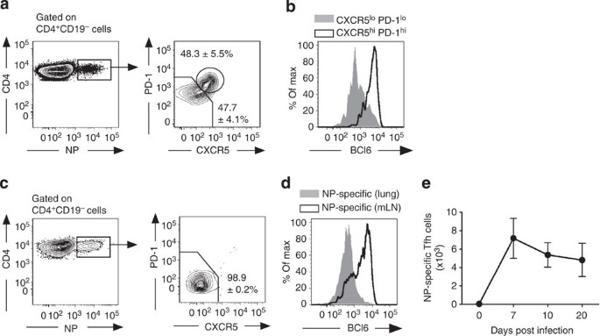Figure 2: Influenza-specific Tfh cells are found in mLN but not the lung. (a–d) B6 mice were infected with PR8 and cells were analysed by flow cytometry on day 10. (a) The frequency of PD-1hiCXCR5hiTfh cells and PD-1loCXCR5loTeff cells in the NP-specific CD4+T cells from the mLN. (b) Bcl6 expression on PD-1hiCXCR5hiand PD-1loCXCR5loNP-specific CD4+T cells. (c) The frequency of PD-1loCXCR5loTeff cells in the NP-specific CD4+T cells from the lung. (d) Bcl6 expression on NP-specific CD4+T cells obtained from the lungs and mLNs. (e) B6 mice were infected with PR8 and the number of NP-specific CD4+Bcl6hiPD-1hiCXCR5hicells in the mLN was calculated at the indicated times. Data are shown as the mean±s.d. (n=4–5 mice per point). Data are representative of three independent experiments. Figure 2: Influenza-specific Tfh cells are found in mLN but not the lung. ( a – d ) B6 mice were infected with PR8 and cells were analysed by flow cytometry on day 10. ( a ) The frequency of PD-1 hi CXCR5 hi Tfh cells and PD-1 lo CXCR5 lo Teff cells in the NP-specific CD4 + T cells from the mLN. ( b ) Bcl6 expression on PD-1 hi CXCR5 hi and PD-1 lo CXCR5 lo NP-specific CD4 + T cells. ( c ) The frequency of PD-1 lo CXCR5 lo Teff cells in the NP-specific CD4 + T cells from the lung. ( d ) Bcl6 expression on NP-specific CD4 + T cells obtained from the lungs and mLNs. ( e ) B6 mice were infected with PR8 and the number of NP-specific CD4 + Bcl6 hi PD-1 hi CXCR5 hi cells in the mLN was calculated at the indicated times. Data are shown as the mean±s.d. ( n =4–5 mice per point). Data are representative of three independent experiments. Full size image To test whether Tregs inhibited the Tfh response to influenza, we infected B6 and FoxP3-DTR mice with influenza, treated them with DT on days 0, 4 and 7 and enumerated NP-specific Tfh and Teff in the mLN on day 10. We found that, although NP-specific CD4 + cells were easily detected in Treg-depleted mice ( Fig. 3a,b ), the frequency of NP-specific CD4 + PD-1 hi CXCR5 hi Tfh cells ( Fig. 3c , top) and NP-specific CD4 + Bcl6 hi cells ( Fig. 3c , bottom) was decreased in the absence of Tregs. As a consequence, the number of NP-specific Tfh cells was dramatically reduced in the mLNs of Treg-depleted mice ( Fig. 3d ). 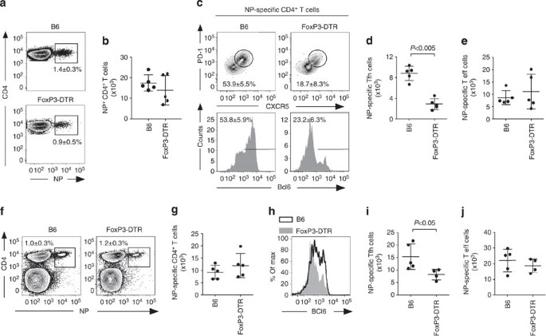Figure 3: Treg depletion compromises influenza-specific Tfh cell responses. (a–e) B6 and FoxP3-DTR mice were infected with PR8, administered DT on days 0, 4 and 7 after infection and the frequency (a) and number (b) of NP-specific CD4+T cells in the mLN was determined by flow cytometry. The frequency of PD-1hiCXCR5hicells (c, top row) and the frequency of Bcl6hicells (c, bottom row) in the NP-specific CD4+T-cell population in the mLN was determined by flow cytometry and the numbers of NP-specific CD4+Bcl6hiPD-1hiCXCR5hicells (d) and NP-specific CD4+Bcl6loPD-1loCXCR5locells (e) in the mLN were calculated. (f,g) B6 and FoxP3-DTR mice were infected with PR8, administered DT on days 0, 4 and 7 after infection and the frequency (f) and number (g) of NP-specific CD4+T cells in the lungs on day 10 were determined by flow cytometry. Data are representative of five independent experiments (mean±s.d of five mice per group).P-values were determined using a two-tailed Student’st-test. (h–j) B6 and FoxP3-DTR mice were infected with PR8, administered DT on days 6 and 10 and the expression of Bcl6 in NP-specific CD4+T cells (h), the number of NP-specific CD4+Bcl6hiPD-1hiCXCR5hicells (i) and the number of NP-specific CD4+Bcl6loPD-1loCXCR5locells (j) was determined in the mLN on day 12. Data are representative of two independent experiments (mean±s.d of four to five mice per group).P-values were determined using a two-tailed Student’st-test. Figure 3: Treg depletion compromises influenza-specific Tfh cell responses. ( a – e ) B6 and FoxP3-DTR mice were infected with PR8, administered DT on days 0, 4 and 7 after infection and the frequency ( a ) and number ( b ) of NP-specific CD4 + T cells in the mLN was determined by flow cytometry. The frequency of PD-1 hi CXCR5 hi cells ( c , top row) and the frequency of Bcl6 hi cells ( c , bottom row) in the NP-specific CD4 + T-cell population in the mLN was determined by flow cytometry and the numbers of NP-specific CD4 + Bcl6 hi PD-1 hi CXCR5 hi cells ( d ) and NP-specific CD4 + Bcl6 lo PD-1 lo CXCR5 lo cells ( e ) in the mLN were calculated. ( f , g ) B6 and FoxP3-DTR mice were infected with PR8, administered DT on days 0, 4 and 7 after infection and the frequency ( f ) and number ( g ) of NP-specific CD4 + T cells in the lungs on day 10 were determined by flow cytometry. Data are representative of five independent experiments (mean±s.d of five mice per group). P -values were determined using a two-tailed Student’s t -test. ( h – j ) B6 and FoxP3-DTR mice were infected with PR8, administered DT on days 6 and 10 and the expression of Bcl6 in NP-specific CD4 + T cells ( h ), the number of NP-specific CD4 + Bcl6 hi PD-1 hi CXCR5 hi cells ( i ) and the number of NP-specific CD4 + Bcl6 lo PD-1 lo CXCR5 lo cells ( j ) was determined in the mLN on day 12. Data are representative of two independent experiments (mean±s.d of four to five mice per group). P -values were determined using a two-tailed Student’s t -test. Full size image In contrast, the number of NP-specific Teff cells was similar in the mLNs of DT-treated B6 and FoxP3-DTR mice ( Fig. 3e ). We also found that the frequency ( Fig. 3f ) and number ( Fig. 3g ) of NP-specific CD4 + T cells (all Teff cells) was similar in the lungs of Treg-depleted and control mice. Taken together, these data suggested that FoxP3-expressing cells promote, rather that inhibit, the influenza-specific Tfh response. We next tested whether Tregs promoted NP-specific Tfh responses beyond the initial priming. Thus, we infected B6 and FoxP3-DTR with influenza, treated them with DT on days 6 and 9 and enumerated NP-specific Tfh cells on day 12. We found that NP-specific CD4 + T cells expressed less Bcl6 ( Fig. 3h ) and that the number of NP-specific Tfh cells was decreased ( Fig. 3i ) in mice depleted of Tregs starting on day 6 after infection. In contrast, Treg depletion starting on day 6 did not affect the number of NP-specific Teff cells ( Fig. 3j ). These results indicated that Treg depletion compromised the maintenance of NP-specific Tfh cells, rather than diverting the differentiation of NP-specific CD4 + T-cell responses towards the Teff pathway. NP-specific Tfh cells are not derived from FoxP3 + precursors Under some circumstances, FoxP3-expressing Tregs can upregulate Bcl6, PD-1 and CXCR5 and downregulate Foxp3, resulting in their differentiation into Tfh cells [30] . In addition, CD4 + T cells may transiently express FoxP3 following activation [33] . Thus, the reduction in NP-specific Tfh cells that we observed in DT-treated FoxP3-DTR mice could be due to the depletion of NP-specific, FoxP3-expressing Tfh precursors. To address this possibility, we first analysed whether NP-specific CD4 + T cells expressed FoxP3. We found that although FoxP3 expression was easily detected in the total CD4 + T-cell population, no FoxP3 expression was detected in either NP-specific CD4 + PD-1 hi CXCR5 hi or NP-specific CD4 + PD-1 lo CXCR5 lo cells on day 10 after infection ( Fig. 4a ). 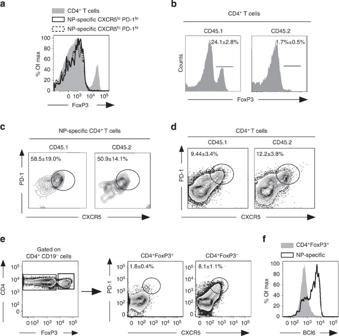Figure 4: Tfh cells do not originate from Foxp3-expressing precursors. (a) B6 mice were infected with PR8 and the expression of FoxP3 on total CD4+T cells NP-specific CD4+PD-1hiCXCR5hiand NP-specific CD4+PD-1loCXCR5locells from the mLN were analysed by flow cytometry on day 10. (b–d) B6 mice were irradiated and reconstituted with a 50:50 mix of BM from B6 (CD45.1) and FoxP3-DTR donors (CD45.2). Reconstituted mice were infected with PR8, administered DT on days 0, 4 and 7 after infection the frequency of CD4+FoxP3+cells (b), the frequency of NP-specific CD4+PD-1hiCXCR5hicells (c) and the frequency of CD4+PD-1hiCXCR5hicells (d) from CD45.1 or CD45.2 donors was determined by flow cytometry. Data are representative of three independent experiments (mean±s.d of four to five mice per group). (e,f) B6 mice were infected with PR8 and the frequency of PD-1hiCXCR5hicells in CD4+FoxP3−or CD4+FoxP3+T cells (mean±s.d of 5 mice per group) (e) and the expression of Bcl6 in NP-specific CD4+cells and CD4+FoxP3+cells (f) were determined by flow cyometry on day 10. All data were obtained after gating on CD19−cells. Data are representative of five independent experiments. Figure 4: Tfh cells do not originate from Foxp3-expressing precursors. ( a ) B6 mice were infected with PR8 and the expression of FoxP3 on total CD4 + T cells NP-specific CD4 + PD-1 hi CXCR5 hi and NP-specific CD4 + PD-1 lo CXCR5 lo cells from the mLN were analysed by flow cytometry on day 10. ( b – d ) B6 mice were irradiated and reconstituted with a 50:50 mix of BM from B6 (CD45.1) and FoxP3-DTR donors (CD45.2). Reconstituted mice were infected with PR8, administered DT on days 0, 4 and 7 after infection the frequency of CD4 + FoxP3 + cells ( b ), the frequency of NP-specific CD4 + PD-1 hi CXCR5 hi cells ( c ) and the frequency of CD4 + PD-1 hi CXCR5 hi cells ( d ) from CD45.1 or CD45.2 donors was determined by flow cytometry. Data are representative of three independent experiments (mean±s.d of four to five mice per group). ( e , f ) B6 mice were infected with PR8 and the frequency of PD-1 hi CXCR5 hi cells in CD4 + FoxP3 − or CD4 + FoxP3 + T cells (mean±s.d of 5 mice per group) ( e ) and the expression of Bcl6 in NP-specific CD4 + cells and CD4 + FoxP3 + cells ( f ) were determined by flow cyometry on day 10. All data were obtained after gating on CD19 − cells. Data are representative of five independent experiments. Full size image To test whether FoxP3 was ever expressed in NP-specific Tfh cells or their precursors, we reconstituted irradiated CD45.1 mice with a 50:50 mix of bone marrow (BM) from CD45.1 donors and FoxP3-DTR donors (CD45.2). Eight weeks post-reconstitution, we infected the chimeric animals with influenza, treated them with DT on days 0, 4 and 7 and enumerated FoxP3 + CD4 + T cells and Tfh cells derived from either the CD45.1-expressing or CD45.2-expressing donors. As expected, DT treatment ablated all of the CD4 + FoxP3 + CD45.2 + cells, but had no effect on the CD4 + FoxP3 + CD45.1 + cells ( Fig. 4b ). In contrast, we found similar frequencies of NP-specific CD4 + CXCR5 hi PD-1 hi Tfh cells derived from both CD45.1 + or CD45.2 + donors ( Fig. 4c ). We observed similar results when we examined the total Tfh pool ( Fig. 4d ). Thus, we concluded that the loss of NP-specific Tfh cells in Treg-depleted mice was not due to the depletion of FoxP3-expressing Tfh cells or FoxP3-expressing precursors of Tfh cells. Following immunization, some Tregs upregulate Bcl6, PD-1 and CXCR5 and continue to maintain FoxP3 expression, resulting in their differentiation into TFR cells [24] , [25] , [34] . Thus, we also tested whether Tregs differentiated into TFR cells following influenza infection. We found only a small percentage of PD-1 hi CXCR5 hi cells in the Foxp3 + CD4 + population ( Fig. 4e ), whereas we found a much higher frequency of PD-1 hi CXCR5 hi cells in the Foxp3 − CD4 + population. Similarly, we found almost no Bcl6 hi cells in the FoxP3 + CD4 + population ( Fig. 4f ). These results demonstrated that TFR cells are not a significant component of the FoxP3 + CD4 + population following flu infection and suggested that the depletion of NP-specific Foxp3 + PD-1 hi CXCR5 hi CD4 + T cells was not the likely cause of the reduced NP-specific Tfh response observed in the DT-treated FoxP3-DTR mice. Normal Tfh and GC B cells responses in the absence of TGF-β Tregs suppress T- and B-cell responses by a variety of mechanisms, including the secretion of the immunosuppressive cytokine, transforming growth factor-β (TGF-β) [35] . To directly test whether TGF-β signalling was important for the development of NP-specific Tfh and GC B cells, we treated B6 mice with control or anti-TGF-β antibody, infected them with influenza and measured NP-specific Tfh cell responses on day 10 after infection. We found that NP-specific CD4 + T cells accumulated similarly in mice treated with anti-TGF-β and control IgG ( Fig. 5a,b ). We also found that NP-specific CD4 + T cells expressed similar amounts of Bcl6, regardless of whether they were from mice treated with anti-TGF-β or control IgG ( Fig. 5c ). Moreover, the frequency of NP-specific CD4 + PD-1 hi CXCR5 hi cells ( Fig. 5d ), and the number of NP-specific CD4 + PD-1 hi CXCR5 hi cells ( Fig. 5e ) was similar in anti-TGF-β treated and control IgG-treated mice. Finally, we found that the number of total PNA hi CD38 lo FAS hi GC B cells ( Fig. 5f ) and NP-specific PNA hi CD38 lo FAS hi GC B cells ( Fig. 5g ) was similar in anti-TGF-β-treated and control mice. Thus, the impaired NP-specific Tfh and GC B-cell responses observed in the absence of Tregs were not due to the loss of TGF-β signalling. 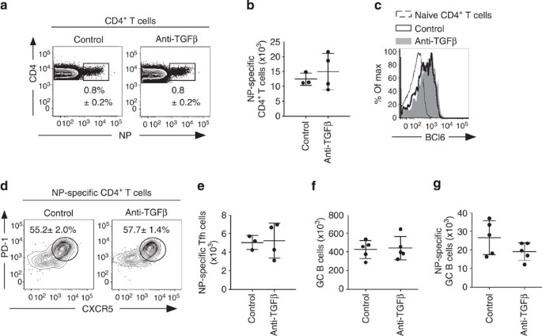Figure 5: TGF-β blockade does not affect influenza-specific Tfh or GC B-cell responses. (a–g) B6 mice were infected with PR8 and were treated with 250 μg of anti-TGF-β or isotype-matched control antibody on days 0 and 5 and the frequency (a) and number (b) of NP-specific CD4+T cells, the expression of Bcl6 on NP-specific CD4+T cells (c), the frequency (d) and number (e) of NP-specific CD4+PD-1hiCXCR5hicells was determined by flow cytometry on day 10 in the mLNs. (f,g) B6 mice were infected with PR8 and treated on days 0 and 5 with 250 μg of anti-TGF-β or control antibody and the number of CD19+PNA+CD38loCD138−GC B cells (f) and the number of NP-specific CD19+PNA+CD38loGC B cells (g) in the mLNs was determined by flow cytometry on day 10. Data are representative of three independent experiments (mean±s.d of four to five mice per group). Figure 5: TGF-β blockade does not affect influenza-specific Tfh or GC B-cell responses. ( a – g ) B6 mice were infected with PR8 and were treated with 250 μg of anti-TGF-β or isotype-matched control antibody on days 0 and 5 and the frequency ( a ) and number ( b ) of NP-specific CD4 + T cells, the expression of Bcl6 on NP-specific CD4 + T cells ( c ), the frequency ( d ) and number ( e ) of NP-specific CD4 + PD-1 hi CXCR5 hi cells was determined by flow cytometry on day 10 in the mLNs. ( f , g ) B6 mice were infected with PR8 and treated on days 0 and 5 with 250 μg of anti-TGF-β or control antibody and the number of CD19 + PNA + CD38 lo CD138 − GC B cells ( f ) and the number of NP-specific CD19 + PNA + CD38 lo GC B cells ( g ) in the mLNs was determined by flow cytometry on day 10. Data are representative of three independent experiments (mean±s.d of four to five mice per group). Full size image Tregs help Tfh cell response to influenza by limiting IL-2 Tregs compete with other T cells for IL-2 and can regulate T-cell responses by IL-2 consumption [16] , [19] , [20] . As excessive IL-2 signalling prevents Bcl6 expression and suppresses the differentiation of Tfh cells [10] , [11] , [12] , [13] , we next tested whether the loss of Tregs resulted in excess IL-2 that prevented the Tfh differentiation. To address this possibility, we first infected B6 and FoxP3-DTR mice with influenza, treated them with DT on days 0, 4 and 7 and determined the frequency of IL-2-producing CD4 + T cells in the mLN on day 10 after infection. We found that the frequency of both IFNγ-producing ( Fig. 6a ) and IL-2-producing ( Fig. 6b ) CD4 + T cells was increased in Treg-depleted mice compared with control animals. 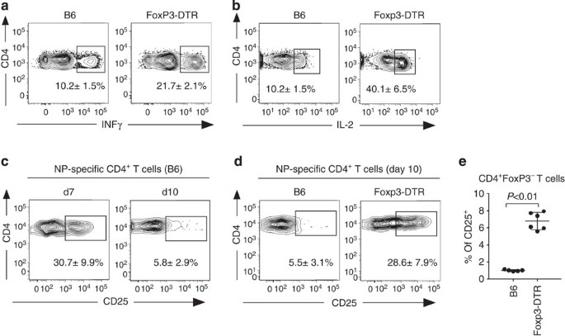Figure 6: Increased IL-2 production and CD25 expression in Treg-depleted mice. (a,b) B6 and FoxP3-DTR mice were infected with PR8, administered DT on days 0, 4 and 7 and, on day 10, cells from the mLN were restimulatedin vitroand the frequencies of IFNγ-producing CD4+cells (a) and IL-2-producing CD4+cells (b) were determined by intracellular staining. (c) B6 mice were infected with PR8 and the frequency of NP-specific CD4+CD25+T cells was determined by flow cytometry in the mLN on days 7 and 10 after infection. (d,e) B6 and FoxP3-DTR mice were infected with PR8, administered DT on days 0, 4 and 7 and the frequency of NP-specific CD4+CD25+cells (d) and the frequency of CD4+CD25+FoxP3−cells (e) was determined by flow cytometry in the mLN on 10 after infection. Data are representative of three independent experiments (mean±s.d. of four to five mice per group).P-values were determined using a two-tailed Student’st-test. Figure 6: Increased IL-2 production and CD25 expression in Treg-depleted mice. ( a , b ) B6 and FoxP3-DTR mice were infected with PR8, administered DT on days 0, 4 and 7 and, on day 10, cells from the mLN were restimulated in vitro and the frequencies of IFNγ-producing CD4 + cells ( a ) and IL-2-producing CD4 + cells ( b ) were determined by intracellular staining. ( c ) B6 mice were infected with PR8 and the frequency of NP-specific CD4 + CD25 + T cells was determined by flow cytometry in the mLN on days 7 and 10 after infection. ( d , e ) B6 and FoxP3-DTR mice were infected with PR8, administered DT on days 0, 4 and 7 and the frequency of NP-specific CD4 + CD25 + cells ( d ) and the frequency of CD4 + CD25 + FoxP3 − cells ( e ) was determined by flow cytometry in the mLN on 10 after infection. Data are representative of three independent experiments (mean±s.d. of four to five mice per group). P -values were determined using a two-tailed Student’s t -test. Full size image Given that CD25 expression is induced in response to IL-2 (refs 36 , 37 ), we next determined whether Treg depletion affected the expression of CD25 on NP-specific CD4 + T cells after influenza infection. We found that more than 30% of the NP-specific CD4 + T cells expressed CD25 on day 7 after infection in B6 mice ( Fig. 6c ), but that only about 5% of the cells continued to express CD25 on day 10. In contrast, nearly 30% of the NP-specific CD4 + T cells continued to express CD25 in Treg-depleted mice on day 10 ( Fig. 6d ). Similarly, the frequency of CD25-expressing cells within the total Foxp3 − CD4 + population was elevated in the absence of Tregs ( Fig. 6e ). Taken together, these results suggest that NP-specific CD4 + T cells receive quantitatively different signals from the IL-2 receptor in control and Treg-depleted mice. To directly determine whether excessive IL-2 signalling was responsible for the loss of Tfh in Treg-depleted mice, we reconstituted irradiated Tcrβδ −/− recipient mice with a 50:50 mix of Cd25 −/− BM (CD45.2) and FoxP3-DTR BM (CD45.1; Fig. 7a ). Because Tregs cannot be produced from C d25 −/− precursors, all the FoxP3 + Tregs in the chimeras developed from the CD45.1-expressing Cd25 +/+ -FoxP3-DTR BM ( Fig. 7b ), whereas the FoxP3 − CD4 + cells developed equally from both donors ( Fig. 7c ). We subsequently infected groups of chimeric mice with influenza, treated them with either DT or PBS on days 0, 4 and 7 and enumerated Tregs, Tfh cells and GC B cells on day 10 in the mLN. We found that Tregs were present only from CD45.1-expressing donors in PBS-treated chimeras ( Fig. 7d,e ), whereas Tregs were not found from either donor in DT-treated chimeras ( Fig. 7d,e ). Consistent with the idea that the loss of Tregs is associated with increased IL-2 signalling, we found that CD25 was expressed by a higher frequency of CD45.1 + NP-specific CD4 + T cells in DT-treated chimeras than in PBS-treated chimeras ( Fig. 7f ). Interestingly, we observed that the number of NP-specific Tfh cells was reduced by about 50% in DT-treated chimeras ( Fig. 7g ), which is about what we expected, as only half of the T cells can respond to IL-2. Importantly, the frequency of NP-specific CD4 + T cells that expressed Bcl6 was reduced only in the CD45.1 + cells from the DT-treated chimeras ( Fig. 7h ). As a result, the number of NP-specific CD4 + PD-1 hi CXCR5 hi Bcl6 hi Tfh cells derived from CD25 +/+ donors was reduced in DT-treated chimeras ( Fig. 7i ), but not in PBS-treated chimeras. Thus, the loss of Tregs preferentially suppresses the development of Tfh that have the ability to respond to IL-2. 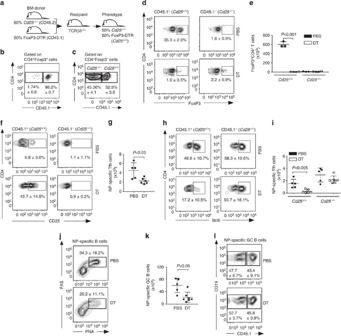Figure 7: Excessive IL-2 signalling after Treg depletion inhibits Tfh cell responses. (a–c) IrradiatedTcrβδ−/−mice were reconstituted with a 50:50 mix of BM fromCd25−/−donors (CD45.2) and FoxP3-DTR donors (CD45.1). Reconstituted mice were infected with PR8 and the percentages of CD45.1+and CD45.1−cells within the CD4+FoxP3+cells (b) and the CD4+FoxP3−T cells (c) determined by flow cytometry on day 10. (d–l) IrradiatedTcrβδ−/−mice were reconstituted with a 50:50 mix of BM fromCd25−/−donors (CD45.2) and FoxP3-DTR donors (CD45.1), infected with PR8, treated with either PBS or DT and the frequency (d) and number (e) of CD4+FoxP3+cells derived from either CD45.1 or CD45.2 donors was determined by flow cytometry on day 10. The frequency of CD4+CD25+in NP-specific cells (f) derived from either CD45.1 or CD45.2 donors was determined by flow cytometry on day 10. The number of total NP-specific CD4+Bcl6hiPD-1hiCXCR5hicells (g) was calculated on day 10. The frequency of CD4+Bcl6hiin NP-specific cells (h) derived from either the CD45.1 or CD45.2 donors was determined on day 10. The number of NP-specific CD4+Bcl6hiPD-1hiCXCR5hicells (i) derived from either the CD45.1 or CD45.2 donors was determined by flow cytometry. The frequency (j) and number (k) of NP-specific CD19+FAS+PNA+GC B cells was determined on day 10. The frequency of NP-specific B cells derived from either the CD45.1 or CD45.2 donors (l) was determined by flow cytometry on day 10. Data are representative of four independent experiments (mean±s.d of four to five mice per group).P-values were determined using a two-tailed Student’st-test. Figure 7: Excessive IL-2 signalling after Treg depletion inhibits Tfh cell responses. ( a – c ) Irradiated Tcrβδ −/− mice were reconstituted with a 50:50 mix of BM from Cd25 −/− donors (CD45.2) and FoxP3-DTR donors (CD45.1). Reconstituted mice were infected with PR8 and the percentages of CD45.1 + and CD45.1 − cells within the CD4 + FoxP3 + cells ( b ) and the CD4 + FoxP3 − T cells ( c ) determined by flow cytometry on day 10. ( d – l ) Irradiated Tcrβδ −/− mice were reconstituted with a 50:50 mix of BM from Cd25 −/− donors (CD45.2) and FoxP3-DTR donors (CD45.1), infected with PR8, treated with either PBS or DT and the frequency ( d ) and number ( e ) of CD4 + FoxP3 + cells derived from either CD45.1 or CD45.2 donors was determined by flow cytometry on day 10. The frequency of CD4 + CD25 + in NP-specific cells ( f ) derived from either CD45.1 or CD45.2 donors was determined by flow cytometry on day 10. The number of total NP-specific CD4 + Bcl6 hi PD-1 hi CXCR5 hi cells ( g ) was calculated on day 10. The frequency of CD4 + Bcl6 hi in NP-specific cells ( h ) derived from either the CD45.1 or CD45.2 donors was determined on day 10. The number of NP-specific CD4 + Bcl6 hi PD-1 hi CXCR5 hi cells ( i ) derived from either the CD45.1 or CD45.2 donors was determined by flow cytometry. The frequency ( j ) and number ( k ) of NP-specific CD19 + FAS + PNA + GC B cells was determined on day 10. The frequency of NP-specific B cells derived from either the CD45.1 or CD45.2 donors ( l ) was determined by flow cytometry on day 10. Data are representative of four independent experiments (mean±s.d of four to five mice per group). P -values were determined using a two-tailed Student’s t -test. Full size image To determine whether Treg depletion differentially affected influenza-specific GC B-cell responses from CD25 +/+ or CD25 −/− donors, we infected chimeric mice with influenza, treated them with DT or PBS on days 0, 4 and 7 and enumerated NP-specific GC B cells on day 10. We found that Treg depletion significantly compromised the accumulation of NP-specific GC B cells ( Fig. 5j,k ). However, the NP-specific GC B-cell population was derived equally from Cd25 +/+ and Cd25 −/− cells in both control and DT-treated mice ( Fig. 7l ). Thus, the ability of B cells to receive IL-2 signals had no impact on their ability to form GCs. Taken altogether, our results indicated that Tregs enhanced influenza-specific Tfh responses by preventing the accumulation of IL-2, which impairs the differentiation of Tfh and indirectly leads to reductions in GC responses. Tregs are well-documented to suppress the activity of both T cells and B cells [14] , [25] , [26] , [32] . However, our data show that overall, Tregs promote, rather than suppress, antigen-specific Tfh and B-cell responses to influenza. The ability of Tregs to promote Tfh responses to influenza is not due to the differentiation of antigen-specific Tfh cells from FoxP3-expressing precursors, as can occur in lymphoid tissues draining the gut [30] . Instead, we find that Tregs indirectly promote influenza-specific Tfh responses by regulating the availability of IL-2 and preventing excessive IL-2 signalling. As IL-2 prevents the differentiation of Tfh cells by preventing Bcl6 expression [10] , [11] , [12] , [13] , the Treg-mediated reduction in IL-2 availability allows more Tfh cells to differentiate and, as a consequence, promotes GC formation. Thus, one of the same mechanisms used by Tregs to suppress effector T-cell responses [19] , [20] , [21] , [23] , IL-2 deprivation, actually enhances Tfh and B-cell responses to influenza. Importantly, these results do not preclude a suppressive function of Tregs in immune responses to influenza infection. In fact, we observe that although the magnitude of the influenza-specific Teff response is not noticeably increased upon Treg depletion, more CD4 T cells produce IL-2 and IFNγ in Treg-depleted mice than in control mice. Similarly, both the magnitude and cytokine-producing ability of influenza-specific CD8 T cells is increased in Treg-depleted mice (not shown). The increased production of IL-2 by effector CD4 and CD8 T cells in Treg-depleted mice is likely one mechanism that increases IL-2 availability. However, Tregs also consume IL-2 via the activity of CD25. Thus, the lack of IL-2 consumption may also contribute to the increased overall availability of IL-2 in Treg-depleted mice. As a result, Treg depletion leads to increased IL-2 production and reduced IL-2 consumption, which promotes effector T-cell differentiation, but paradoxically reduces the numbers of Tfh, and by extension, impairs the ability of B cells to form GC. The idea that Tregs can enhance Tfh and B-cell responses to influenza is at odds with their well-known ability to suppress autoreactive Tfh and B cells [24] , [25] , [28] , [34] . For example, mice [32] , [38] and humans [39] , [40] , [41] , [42] that lack Tregs due to natural or gene-targeted mutations of FoxP3 develop severe autoimmune disease, including the spontaneous accumulation of autoreactive Tfh cells and GCs [25] . However, it is important to distinguish between the ability of Tregs to suppress the activation of autoreactive T cells and their ability to alter the differentiation pathway of CD4 T cells responding to foreign antigens. For example, when Tregs are depleted or congenitally absent, autoreactive cells become activated. Although the depletion of Tregs obviously abrogates their ability to regulate IL-2 availability, we would expect that IL-2 is sufficiently limiting in this scenario to allow the differentiation of autoreactive T cells into Tfh cells even in the absence of Treg. Thus, Tfh and GC B cells accumulate over time in Treg-deficient individuals. Interestingly, T cells from autoimmune mice and patients make less IL-2 than their normal counterparts [43] and perhaps allow the more efficient differentiation of autoreactive Tfh cells. Conversely, treatment of autoimmune mice and humans with IL-2 improves disease in some cases [44] , [45] , [46] , [47] , possibly by increasing Treg numbers or activity, but perhaps also by limiting Tfh differentiation. Thus, the involvement of IL-2 and Tregs in the regulation of autoreactive Tfh and GC reactions is complex and somewhat paradoxical. Although Tregs obviously prevent the initial activation of autoreactive cells, this suppressive activity must be overcome in response to foreign antigens. For example, Treg activity is suppressed by cytokines like IL-6 during the acute inflammatory response that occurs following influenza infection [48] . As a result, the initial activation of influenza- specific CD4 T cells likely proceeds in the absence of Treg suppressor activity. Nevertheless, Tregs will likely continue to consume IL-2, leading to an enhanced differentiation of influenza-specific CD4 T cells into Tfh cells, which subsequently promote the expansion of influenza-specific GCs. Other investigators have observed a similar decrease in antigen-specific B-cell responses following Treg depletion [24] , [31] . For example, mucosal IgG and IgA responses to protein antigens and cholera toxin are reduced following Treg depletion [31] . Another study shows that although the number of total GC B cells is increased in DT-treated FoxP3-DTR mice following immunization with NP-KLH, the number of NP-specific GC B cells is actually decreased [24] . Although the mechanism underlying the decreased GC responses was not determined in these studies, we suspect that increased IL-2 availability is a likely cause. Despite their ability to enhance Tfh differentiation via the control of IL-2 availability, Tregs also have mechanisms that directly suppress B-cell responses. For example, Tregs can directly prevent B-cell proliferation [27] , [28] , inhibit antibody production [25] and in some cases, kill activated B cells via a perforin and granzyme B-dependent mechanism [27] . These mechanisms are likely to be used by TFR cells in the GC, where they suppress ongoing GC reactions [24] , [25] , [34] . Interestingly, we observed very few TFR cells following influenza infection, perhaps because the elevated IL-2 response at the peak of influenza infection prevents Tregs from upregulating Bcl6 and differentiating into TFR cells. Given the scarcity of TFR cells in our experiments, it makes sense that their ability to directly suppress GC reactions is minimal. Thus, the ability of conventional Tregs to consume IL-2 and promote Tfh differentiation may be more noticeable following influenza infection than it is following immunization with protein antigens. Another explanation for why the suppressive activity of Tregs on GC responses is more evident in some studies may be the amount of IL-2 generated during a particular immune response. If the amount of IL-2 generated following influenza infection is relatively high compared with the amount generated following immunization with protein antigens, then the ability of Tregs to regulate IL-2 availability may be more important in the context of influenza infection. For example, when IL-2 is abundant, Tfh differentiation will be suppressed and the ability of Tregs to regulate IL-2 availability will be important to overcome the negative effect of IL-2. In contrast, when IL-2 is scarce, Tfh differentiation will not be impeded and the ability of Tregs to regulate IL-2 will not make a difference, allowing the suppressive activity of Tregs to be more noticeable. Thus, the ability of Tregs to promote Tfh and GC responses by regulating IL-2 may be context dependent. The activity of Tregs is also likely to be location dependent. Following initial encounter with antigen, some activated CD4 + T cells upregulate CXCR5 and migrate to the interfollicular zone, where they further upregulate Bcl6 and complete the Tfh differentiation programme [49] , [50] , [51] , [52] . Thus, one way by which Tregs might promote Tfh cell development is by limiting IL-2 availability within the interfollicular area, which would in turn allow preTfh cells to maintain Bcl6 expression. Thus, placement of Tregs near the B follicles would be required for their ability to promote Tfh cell responses, an idea that is consistent with the presence of FoxP3 + cells in the proximity of the T:B border [26] , [28] , [29] , but at odds with our results showing that Tregs do not express CXCR5 following influenza infection. Interestingly, stromal cells within the interfollicular area also produce CXCL9 and attract CXCR3-expressing T cells to the interfollicular and medullary zones [53] . Thus, Tregs may gain access to the interfollicular zone by a CXCR3-dependent mechanism. In agreement with this view, Tregs upregulate CXCR3 after influenza infection and other type 1 inflammatory responses [14] , [54] . In addition, Tregs may regulate IL-2 availability in the T-cell area, which may prevent preTfh from upregulating Bcl6 and, at the same time, favour CD8 T-cell expansion. Collectively our findings offer a new perspective for how Tfh cell development is regulated in vivo and open new roads in the study of non-suppressive functions of Tregs in the control of the immune response to infection. Mice and infections C57BL/6 (B6), B6.129S4- Il2ra tm1Dw/J ( Cd25 −/− ), B6. IgH a .Thy-1 a .Ptrpc a (CD45.1) and B6.129P2- Tcrβ tm1Mom Tcrd tm1Mom ( Tcrβδ −/− ) mice were originally obtained from Jackson Laboratories and were bred in the University of Alabama at Birmingham animal facility. B6.129S6- Foxp3 tm1DTR (FoxP3-DTR) mice were originally obtained from Dr. Alexander Rudensky (Memorial Sloan-Kettering Cancer Center). B6.129S6- Foxp3 tm1DTR -CD45.1 + mice were generated by crossing FoxP3-DTR mice with CD45.1 mice. Influenza virus infections were performed intranasally with 500 egg infectious units of A/PR8/34 (PR8) in 100 μl of PBS. Eight-week-old males were used for all the experiments described. BM chimeras and in vivo treatments BM chimeric mice were generated by lethally irradiating the indicated recipient mice with 950 Rads from an X-ray source delivered in two equal doses administered 4–5 h apart. Following irradiation, mice were intravenously injected with 5 × 10 6 total BM cells and allowed to reconstitute for 8–10 weeks before influenza infection. In indicated experiments, experimental animals received an intraperitoneal injection of 50 μg kg −1 of diphtheria toxin (DT; Sigma) at the indicated time points. In some experiments, mice were treated intraperitoneally with 250 μg of anti-TGFβ antibody (clone 1D11.16.8; Bioxcell) or isotype-matched control antibody (MOPC-21; Bioxcell). All experimental procedures involving animals were approved by the University of Alabama Institutional Animal Care and Use Committee and were performed according to guidelines outlined by the National Research Council. Cell preparation and flow cytometry Cell suspensions from mLNs were prepared by passing tissues through nylon mesh. Lungs were cut into small fragments and digested for 45 min at 37 °C with 0.6 mg ml −1 collagenase A (Sigma) and 30 mg ml −1 DNAse I (Sigma) in RPMI-1640 medium (GIBCO). Digested lungs were mechanically disrupted by passage through a wire mesh. Cells from lungs and mLNs were resuspended in 150 mM NH4Cl, 10 mM KHCO3 and 0.1 mM EDTA for 5 min to lyse red cells. Cell suspensions were filtered through a 70 mm nylon cell strainer (BD Biosciences), washed and resuspended in PBS with 5% donor calf serum and 10 mg ml −1 FcBlock (2.4G2; BioxCell) for 10 min on ice before staining with fluorochrome-conjugated antibodies or tetramer reagents. Fluorochrome-labelled anti-CD45.1 (clone A20, dilution 1/400), anti-CD45.2 (clone 104, dilution 1/400), anti-PD-1 (clone J43, dilution 1/100), anti-FoxP3 (clone FJK-16s, dilution 1/200), anti-CD19 (clone 1D3, dilution 1/200), anti-CD138 (clone 281.2, dilution 1/500) were all from eBioscience. Anti-CD8α (clone 53-6.7 dilution 1/200), anti-Bcl6 (clone K112.91, dilution 1/50), anti-CXCR5 (clone 2G-8, dilution 1/50), anti-CD4 (clone RM4-5, dilution 1/200), anti-CD95 (clone RM4-5, dilution 1/500), anti-IL-2 (clone JES6-6H4, dilution 1/200) and anti-CD25 (clone PC61, dilution 1/200) were from BD Biosciences. Peanut agglutinin (PNA) was obtained from Sigma (L7381; Sigma) and conjugated with FITC or Pacific Blue. The IA b NP 311–325 MHC class II tetramer was obtained from the NIH Tetramer Core Facility and used at a 1/100 dilution. To generate the NP-tetramer preparation for detection of influenza-specific B cells, the coding sequence of NP from the A/PR8/34 virus was synthesized in frame with the coding sequence for a 15 amino acid biotinylation consensus site (Schatz) on the 3′ end (GeneArt, Regensburg, Germany). The modified NP sequence was then cloned in frame to the 6X His tag in the pTRC-His2c expression vector (Invitrogen, Carlsbad, CA) and expressed in E. coli strain Ultra BL21 (DE3; EdgeBio, Gaithersburg, MD). The modified NP-protein was purified by FPLC using a HisTrap HP Column (GE Healthcare). Purified protein was biotinylated by addition of Biotin-protein ligase (Avidity, Aurora, CO) and tetramerized with PE-labelled streptavidin (Prozyme, Hayward, CA). Labelled tetramers were purified by size exclusion on a HiPrep 16/60 Sephacryl S-300 column (GE Healthcare, Piscataway, NJ).Dead cell exclusion was performed using 7-AAD (Biolegend). For detection of IL-2-producing cells, single-cell suspensions were stimulated with PMA (5 ng ml −1 ) and calcium ionophore (1.25 μM) in the presence of Brefeldin-A (10 mg ml −1 ) for 3 h. Cells were then surface stained, fixed in 4% paraformaldehyde and permeabilized with 0.1% saponin before staining with anti-IL-2 antibody (JES6-6H4). Intracellular staining for Bcl6 (K112.91) and Foxp3 (FJK-16s), were performed using the mouse regulatory T-cell staining kit (eBioscience) following manufacturer’s instructions. Flow cytometry was performed using a FACSCanto II (BD Biosciences). Statistical analysis The statistical significance of differences in mean values was analysed using a two-tailed Student’s t -test. P -values <0.05 were considered statistically significant. How to cite this article: León, B. et al. FoxP3 + regulatory T cells promote influenza-specific Tfh responses by controlling IL-2 availability. Nat. Commun. 5:3495 doi: 10.1038/ncomms4495 (2014).